Three-dimensional nanonetworks for giant stretchability in dielectrics and conductors The realization of levels of stretchability that extend beyond intrinsic limits of bulk materials is of great importance to stretchable electronics. Here we report large-area, three-dimensional nano-architectures that achieve this outcome in materials that offer both insulating and conductive properties. For the elastomer poly(dimethylsiloxane), such geometries enhance the stretchability and fracture strain by ~62% and ~225% over the bulk, unstructured case. The underlying physics involves local rotations of narrow structural elements in the three-dimensional network, as identified by mechanical modelling. To demonstrate the applications of three-dimensional poly(dimethylsiloxane), we create a stretchable conductor obtained by filling the interstitial regions with liquid metal. This stretchable composite shows extremely high electrical conductivity (~24,100 S cm −1 ) even at strains >200%, with good cyclic properties and with current-carrying capacities that are sufficient for interconnects in light-emitting diode systems. Collectively, these concepts provide new design opportunities for stretchable electronics. Stretchable electronic materials enable classes of applications such as electronic eye cameras [1] , artificial skins [2] , flexible sensors [3] , and actuators [4] that cannot be achieved using conventional, wafer-based technologies. One of the key technical challenges is in the development of materials that can offer the electronic properties of established inorganic materials but also can endure large-strain (>1%), repeated deformations without changes in their characteristics. In most cases, the intrinsic material properties, such as yield strength, Young's modulus, Poisson's ratio, and so on, govern the mechanics. Recently, several approaches have been proposed to improve the stretchability beyond these limits; among these, two appear particularly promising. One exploits pre-stretching of a compliant substrate before bonding thin, stiff inorganic films, either uniformly or at strategic locations. Releasing the pre-strain leads to compression in the films and the corresponding formation of 'wavy' microstructures by the processes of buckling [5] . The other uses net-shaped flexible films with macroscopically perforated holes [6] . Stretchability of conductive elastomers can be extended up to ~140% (ref. 7 ) by perforating, hot-rolling, and the use of a low elastic modulus substrate [8] . A disadvantage is that the stretching range in such two-dimensional structures is limited by the relatively low density of in-plane holes that can be accommodated, in a practical sense, at the millimeter scale. Here we demonstrate a method that significantly improves the stretchability, and the range of design choices, by introducing perforations in full three-dimensional (3D) nanostructured forms, using a process that can easily be scaled to large areas (~625 mm 2 for results reported here). Such 3D net-shaped nanostructures in the elastomer poly(dimethylsiloxane) (PDMS) significantly improve the stretchability (by ~62%) compared with solid films made of the same material, owing to 3D rotations of elastic bridging elements when the structure is stretched. At the same time, the fracture strain is increased by more than ~200%. These enhancement mechanisms are identified quantitatively by theoretical modelling and verified by finite element analysis (FEA), both of which agree well with experimental results. To demonstrate the practical value of such strategies, we build highly stretchable conductors by infilling a liquid-phase eutectic gallium–indium (EGaIn) alloy into the interconnected, 3D porous channels in the structured PDMS. The composite results in extremely high electrical conductivity of ~24,100 S cm −1 at 220% strain without severe deterioration during the many cycles of stretching-releasing. To the best of our knowledge, these values exceed those of other reported stretchable conductors. The 3D nano-architectures and the underlying mechanisms lead to new classes of stretchable materials, for potential use in various electronic and optoelectronic devices, as we demonstrate through interconnected arrays of light-emitting diodes (LEDs). 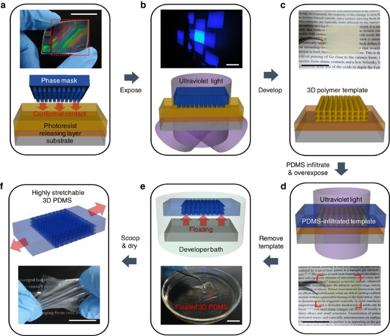Figure 1: Schematic illustration of fabrication procedures to produce 3D PDMS. (a) Conformal contact of a PDMS phase mask against a film of a positive-tone photoresist. (b) Generation of complex 3D distributions of intensity in the photoresist by interference of ultraviolet light (wavelength~355 nm) diffracted by passage through the mask. (c) Washing away the exposed soluble regions using water-based developing solution. (d) Infiltration of PDMS prepolymer into the 3D template, followed by a second flood exposure. (e) Removal of the 3D template and releasing layer (hard-baked photoresist) in a developer bath. (f) Retrieving the floating PDMS membrane and drying it with a stream of air. Scale bar, 2 cm. Fabrication of 3D PDMS Figure 1 illustrates a fabrication route to net-shaped 3D periodic elastomers that uses an optically patterned 3D nanostructure as a template. The process begins with 3D patterning of positive-tone photoresists by proximity-field nanopatterning (PnP) [9] , [10] , [11] , [12] . PnP is an advanced 3D nanofabrication technique that involves a single-step exposure through a conformal phase mask. The mask used here involves surface relief structures consisting of cylindrical posts of diameter of 480 nm, periodicity of 600 nm, and height of 420 nm ( Supplementary Fig. S1 ). Large-area, highly reliable fabrication of various hierarchical 3D nanostructures can be achieved by using large-size phase masks and the PnP technique. The whitish 3D nanostructure, shown in Fig. 1c (which, to date, corresponds to the largest 3D nanostructure patterned by PnP), serves as a template to produce the 3D elastomer. A key advance over previous work is the replacement of conventional 3D resists (e.q. SU-8, Microchem) [13] , which require harsh removal conditions such as high-temperature burning (~500 °C) or plasma etching [14] , with a positive-tone resist (AZ 9260, Clariant). The positive-tone resist can be easily removed by buffered aqueous solution of KOH after infiltration of PDMS, without causing damage to the 3D nano-architecture. When the 3D structure is filled with PDMS, it becomes transparent ( Fig. 1d ) owing to approximate index matching between AZ 9260 and PDMS (refractive indices ~1.6 and ~1.4, respectively). A second flood exposure renders the original template and the releasing layer (hard-baked AZ 9260) soluble by a developer (AZ 400 K, 1:4 dilution of buffered KOH, Clariant). The 3D nanostructured PDMS film with a residual layer of solid PDMS (thickness of the residual layer varies with different preparation condition; Supplementary Fig. S2 ) can then be released from the glass supporting substrate into the developer. A thick slab of PDMS can be used to retrieve the resulting free-standing sheet of 3D PDMS ( Fig. 1e,f ). Figure 1: Schematic illustration of fabrication procedures to produce 3D PDMS. ( a ) Conformal contact of a PDMS phase mask against a film of a positive-tone photoresist. ( b ) Generation of complex 3D distributions of intensity in the photoresist by interference of ultraviolet light (wavelength~355 nm) diffracted by passage through the mask. ( c ) Washing away the exposed soluble regions using water-based developing solution. ( d ) Infiltration of PDMS prepolymer into the 3D template, followed by a second flood exposure. ( e ) Removal of the 3D template and releasing layer (hard-baked photoresist) in a developer bath. ( f ) Retrieving the floating PDMS membrane and drying it with a stream of air. Scale bar, 2 cm. Full size image Most positive-tone resists have high absorption coefficients, which restricts the maximum thicknesses that can be utilized in the PnP process to ~3 μm (refs 15 , 16 ). This limitation can be overcome by the unique optical properties of DNQ-based resists. In particular, this resist system chemically converts into indene-carboxylic acid photoproducts under ultraviolet light, resulting in reduced absorption with increasing exposure time (that is, photo-bleaching effect) [17] ( Fig. 2a ). Accordingly, the achievable thicknesses of 3D patterns increase with exposure dose. However, we note that the use of large doses may result in overexposure at the top of the resist. During development, this can lead to damaged 3D structures near the top and a porosity gradient along the ultraviolet penetration depth. To avoid these problems, exposure time, developing time and resist thickness must be carefully controlled. The structures that result after development become more opaque with increasing exposure dose, because the 3D structure scatters more light as the thickness of the patterned structure increases ( Fig. 2b ) [10] . Cross-sectional scanning electron microscope (SEM) images confirm this effect ( Fig. 2c, d ). Thick 3D structures (~12 μm), containing periodic multilayers, can be fabricated at the exposure dose of ~450 mJ cm −2 . Measured values of the extinction coefficients as a function of dose ( Supplementary Fig. S3 ) and the corresponding light propagation analysed by FEA further explain the phenomena ( Supplementary Fig. S4 ). Over-developing exposes the surfaces of the 3D structures, to reveal successful inner-layer patterning, with results that are consistent with electromagnetic simulations using GSolver (Grating Solver Development) ( Fig. 2e,f ). 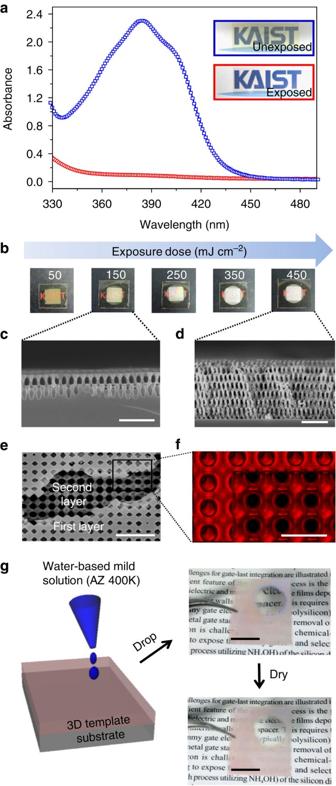Figure 2: Fabrication of 3D periodic templates using thick positive-tone photoresists. (a) Reduction in optical absorption in the DNQ-based photoresist film (AZ 9260, Clariant) induced by photoexposure (Blue open squares: unexposed photoresist film, red open circles: exposed photoresist film). (b) Change in transparency of 3D patterned films with increasing exposure dose. (c) Cross-sectional SEM image of a AZ 9260 film patterned using an exposure dose of ~150 mJ cm−2. Scale bar (also ind,e), 3 μm. (d) Cross-sectional SEM image of a AZ 9260 film patterned using the exposure dose of ~450 mJ cm−2. (e) Top-view SEM image of the top surface of the 3D polymer template after removing part of the first layer. (f) Optical simulations of expected 3D structures, performed by rigorous coupled wave analysis. Scale bar 1 μm. (g) Removal of AZ 9260 templates by acqueous basic solution (AZ 400 K developer, Clariant). Scale bar, 1 cm. Figure 2g shows easy removal of the patterned AZ 9260 by a water-based developer, which does not swell, dissolve or distort soft organic materials such as PDMS [18] ( Supplementary Fig. S5 ). Taken together, these properties make this type of resist ideal for present purposes. Figure 2: Fabrication of 3D periodic templates using thick positive-tone photoresists. ( a ) Reduction in optical absorption in the DNQ-based photoresist film (AZ 9260, Clariant) induced by photoexposure (Blue open squares: unexposed photoresist film, red open circles: exposed photoresist film). ( b ) Change in transparency of 3D patterned films with increasing exposure dose. ( c ) Cross-sectional SEM image of a AZ 9260 film patterned using an exposure dose of ~150 mJ cm −2 . Scale bar (also in d , e ), 3 μm. ( d ) Cross-sectional SEM image of a AZ 9260 film patterned using the exposure dose of ~450 mJ cm −2 . ( e ) Top-view SEM image of the top surface of the 3D polymer template after removing part of the first layer. ( f ) Optical simulations of expected 3D structures, performed by rigorous coupled wave analysis. Scale bar 1 μm. ( g ) Removal of AZ 9260 templates by acqueous basic solution (AZ 400 K developer, Clariant). Scale bar, 1 cm. Full size image Highly stretchable 3D PDMS Vacuum-assisted infiltration provides a route to complete filling of PDMS prepolymer into the sub-micron pores of the 3D templates [15] . Spin-casting follows the infiltration to flatten the surface of the sample. The speed of spin-casting (1,000 to 7,000 r.p.m.) controls the residual thickness of solid PDMS (portion of the prepolymer outside the 3D template, on top). In the following, the thickness of the 3D PDMS is fixed at 12 μm, while the total film thickness ranges from 15 to 90 μm (that is, residual solid layer is 3~78 μm; Supplementary Fig. S6 ). The curing temperature of PDMS was fixed at 60 °C to ensure sufficient crosslinking of polymer chains. Relatively thin 3D PDMS, inversely replicated from the template, experiences severe bending forces because of its high porosity and osmotic pressure during drying immediately after retrieval from the developer. Conformal backing layers of unpatterned PDMS provide mechanical support, for manipulation in a way that minimizes unwanted deformations ( Fig. 3a ). In this way, the 3D PDMS maintains its open porous structures without any distortion or collapse of the interconnected features. The coverage of 3D structures is not limited to bulk volumes, but can also be realized as line or arbitrary shapes by using a superimposed multiple-mask system or performing additional patterning ( Supplementary Fig. S7 ) [19] , [20] . The optical image of a folded 3D PDMS film with line patterns is shown in Fig. 3b . 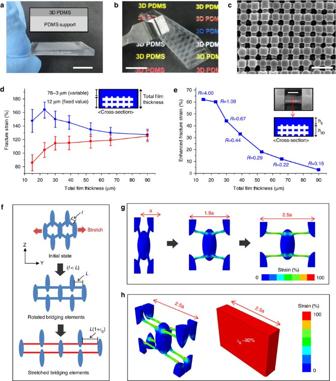Figure 3: Mechanical properties of 3D PDMS. (a) Optical image of a supported 3D PDMS film. Scale bar, 1 cm. (b) Optical image of a folded 3D PDMS film with line patterns. Scale bar, 1 cm. (c) Top-view SEM image of net-shaped 3D PDMS. Scale bar, 1 μm. (d) Comparison of fracture strain between 3D PDMS (blue-filled circles) and solid PDMS (red-filled squares) for various thicknesses. (e) Comparison of extended stretchability for different ratios of thickness of the 3D layer to that of the solid film (R=h3D/hs). Inset: optical image of 3D PDMS attached on the customized tensile tester. Scale bar, 1 cm. (f) Rotation mechanism of the 3D PDMS under stretching along Y-direction, projected in the Y-Z plane. (g) Strain distribution obtained by FEA for the unit cell of 3D PDMS stretched by 90% (middle) and 150% (right). (h) Comparison of strain distributions between 3D PDMS (left) and solid PDMS (right) under 150% stretching. Figure 3c shows a top-view SEM image of 3D PDMS. Figure 3: Mechanical properties of 3D PDMS. ( a ) Optical image of a supported 3D PDMS film. Scale bar, 1 cm. ( b ) Optical image of a folded 3D PDMS film with line patterns. Scale bar, 1 cm. ( c ) Top-view SEM image of net-shaped 3D PDMS. Scale bar, 1 μm. ( d ) Comparison of fracture strain between 3D PDMS (blue-filled circles) and solid PDMS (red-filled squares) for various thicknesses. ( e ) Comparison of extended stretchability for different ratios of thickness of the 3D layer to that of the solid film ( R = h 3D / h s ). Inset: optical image of 3D PDMS attached on the customized tensile tester. Scale bar, 1 cm. ( f ) Rotation mechanism of the 3D PDMS under stretching along Y-direction, projected in the Y-Z plane. ( g ) Strain distribution obtained by FEA for the unit cell of 3D PDMS stretched by 90% (middle) and 150% (right). ( h ) Comparison of strain distributions between 3D PDMS (left) and solid PDMS (right) under 150% stretching. Full size image The resulting 3D nano-architectures in PDMS offer superior levels of stretchability. We identify two important features of the mechanics from the experimental results ( Fig. 3d ). The first is that PDMS films with 3D nanostructures exhibit fracture strains significantly higher than those of solid PDMS films with the same thickness. In other words, 3D periodic networks enhance the fracture limits. The second is that 3D PDMS films show systematically different mechanical behaviour as the overlying solid film thickness decreases. In particular, the 3D PDMS shows increasing fracture strain with decreasing film thickness, whereas solid PDMS typically shows the opposite trend [21] . The stress-strain curves support these experimental results ( Supplementary Fig. S8 ). Once the 3D PDMS reaches breaking point, fracture occurs abruptly. The level of enhancement in stretchability (compared with solid PDMS) significantly increases as the total film thickness ( Fig. 3e ) decreases by reducing the overlayer thickness, that is, as the ratio R of the thickness of the 3D layer to that of the solid layer varies from 0.15 to 4. This effect becomes increasingly dominant as R increases. When R is low (<0.2), the elastic modulus of 3D PDMS is similar to that of solid PDMS. As R increases, the elastic modulus of 3D PDMS is significantly lower than that of solid PDMS at the same film thickness. When R is greater than 1, the elastic modulus of 3D PDMS is ~22% of that of solid PDMS. The curing temperature also influences the mechanical properties, because the degree of PDMS vulcanization heavily depends on this temperature ( Supplementary Fig. S9 ). Elastomers typically have high flexibility and stretchability when cured at low temperatures [22] . The 3D PDMS cured at room temperature shows maximum stretchability of ~225%, which corresponds to the highest value reported for PDMS ( Supplementary Movie S1 for the stretching test of solid PDMS and solid PDMS). Enhancement mechanism An analytical mechanics model, validated by FEA, is developed to identify the mechanism of these enhancements. Although mechanical simulations for large compressive deformation in 2D-ordered porous polymers have been studied [23] , deformation mechanics of 3D-ordered porous elastomers under stretching is not well-known. The symmetry of 3D polymer structure fabricated from PnP is similar to body-centred tetragonal with sub-micron lattice parameters [20] . The shape and geometry of resulting 3D PDMS structures take the inverse form of the original template (see Supplementary Fig. S10 for detailed visualizations and optical simulations on the geometry). As a result, a unit cell of the 3D PDMS consists of ellipsoids (prolate spheroid) with polar radius A and equatorial radius B , respectively ( Supplementary Fig. S11 ). The ellipsoids are packed in a body-centred tetragonal Bravais lattice with square base 2 W ×2 W and height 2 H , and interconnected with bridging elements of length L . The length L is defined as the surface-to-surface distance between two adjacent ellipsoids along the line segment between their origins, and is related to the above geometric parameters by The projection of L into the stretching direction ( y axis, see Supplementary Fig. S11 for direction definitions) is l , as shown in Fig. 3f (where everything is projected into the y – z plane). When the 3D PDMS is stretched, the bridging elements first rotate to the direction of stretching, to accommodate the deformation, which offers an longation of 2·( L - l ) for each unit cell. The strain at this stage mainly involves bending strain, which is small compared with the large stretching that follows. Further stretching mainly appears in the bridging elements, because they have much smaller cross-sectional area (and thus smaller tensile stiffness) than the ellipsoids. Each bridging element can be stretched to a length of L ·(1+ ε s ) before fracture occurs, where the ε s is the fracture strain for solid PDMS. Therefore, the fracture strain for 3D PDMS is This simple model shows that slender unit cell (large H / W ) and relatively small ellipsoids (large H / A and H / B , or the structure being more porous) enhance the stretchability of the 3D PDMS [7] . For experimental data of W =250 nm, H =950 nm, A =500 nm, B =200 nm, and ε s =85% ( Fig. 3d , solid PDMS made at the spin-speed of 7,000 r.p.m. ), equation (2) gives ε 3D =149%, which agrees well with experimental result of 147% ( Fig. 3d ). For, ε s =160%, obtained by curing at room temperature, equation (2) gives ε 3D =219%, which is consistent with experimental result of 225%. Fig. 3g shows FEA results for 3D PDMS under stretching. For 90% strain, the bridging elements rotate to the stretching direction to accommodate the deformation, resulting in strain of only about 20% in the bridging elements; further stretching to 150% significantly increases the strain in the bridging elements to about 70%. During the entire stretching, the bridging elements rotate and stretch to accommodate almost all of the deformation, while the strain in the ellipsoids remains small. The FEA results in Fig. 3g also show that 150% stretch induces a uniform true strain of 92% in the solid PDMS, while the 3D PDMS has strain larger than 90% only in very small, localized regions (small, red area in Fig. 3h ). Consequently, the statistically possible number of fracture points in 3D PDMS during stretching is significantly fewer than that of solid PDMS. High-performance 3D stretchable conductor The high stretchability of 3D PDMS makes it an attractive alternative to solid PDMS as an insulating substrate in stretchable electronics, and potentially as interlayer dielectrics as well. Furthermore, the open spaces can be exploited to achieve composite materials with distinct electronic properties [24] . For example, 3D PDMS can be made electrically conductive by filling conductive materials into the continuous, interconnected channels of its 3D pores. A stretchable conductor, which consists of liquid metal (EGaIn) enclosed in the elastomeric channels at room temperature, is created by sandwiching two thin (~23 μm) 3D PDMS films. The EGaIn can be smoothly injected into 3D channels along the plasma-treated surfaces with vacuum-assistance. The colour of EGaIn is changed from bright silver to whitish gray owing to light scattering after successful filling. 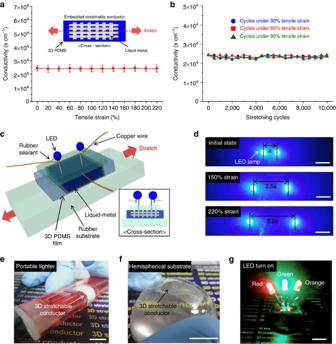Figure 4: Electrical robustness of 3D stretchable conductor and its demonstration through LED applications. (a) Conductivity of embedded stretchable conductors under stretching up to ~220%. (b) Conductivity after cyclic stretching-releasing of various strains. (c) Schematic illustration of LED devices on stretchable conductors. (d) Successful operation under stretching up to ~220%. (e) Conformally attached stretchable conductors on the portable lighter. (f) Conformally attached stretchable conductors on a hemispherical substrate (g) Realization of LED arrays (Red, green, orange colours) using 3D stretchable conductors on the hemispherical substrate (f). Scale bar, 1 cm. Figure 4 summarizes the electrical properties of the resulting composite and its practical demonstration in a simple connection of LEDs. This system shows extremely high electrical conductivity (~24,100 S cm −1 ), comparable to the intrinsic conductivity of EGaIn. The conductivity is invariant during the entire stretching process, owing to the ability of the fluid-phase EGaIn to follow any changes in the shape of the stretched 3D PDMS, and maintain continuous conduction pathways through the porous network ( Fig. 4a ) ( Supplementary Fig. S12a for the conductance change under stretching). The conductivity of ~24,100 S cm −1 at 220% strain represent improvements on previous results for stretchable conductors ( Supplementary Fig. S12b ). The slight decrease in stretchability (~5%) compared with non-conductive 3D PDMS results from the increased portions of solid PDMS around the perimeter, for sealing the EGaIn. Cyclic tensile tests at various strains are shown in Fig. 4b . The conductivity remains nearly the same even after 10,000 cycles of 90% strain, thereby demonstrating the mechanical robustness of this system. This strategy overcomes major weakness of conventional stretchable conductors, which have a trade-off relationship between stretchability and conductivity [25] . Figure 4: Electrical robustness of 3D stretchable conductor and its demonstration through LED applications. ( a ) Conductivity of embedded stretchable conductors under stretching up to ~220%. ( b ) Conductivity after cyclic stretching-releasing of various strains. ( c ) Schematic illustration of LED devices on stretchable conductors. ( d ) Successful operation under stretching up to ~220%. ( e ) Conformally attached stretchable conductors on the portable lighter. ( f ) Conformally attached stretchable conductors on a hemispherical substrate ( g ) Realization of LED arrays (Red, green, orange colours) using 3D stretchable conductors on the hemispherical substrate (f). Scale bar, 1 cm. Full size image The potential applications for 3D stretchable conductors include stretchable antennas, wearable keypads and flexible sensors [26] , [27] , [28] , [29] , [30] , [31] . We demonstrate a simple prototype that consists of commercial LED lamps integrated with and interconnected by the 3D stretchable conductor. Figure 4c shows a schematic illustration of the set-up (see Supplementary Fig. S13 for the real image of the set-up on stretching tester). Two LED lamps are installed near opposite ends of the stretchable conducting layer, and connected through the 3D stretchable conducting layer. The LED lamps are turned on when the applied voltage is greater than 2.3 V ( Supplementary Fig. S14 ) and survive after stretching up to ~220% ( Fig. 4d ). The brightness does not degrade even beyond ~220% because of the electrical and mechanical robustness of embedded stretchable conductor. The illumination power of a LED lamp integrated into the 3D stretchable conductor is comparable to that of a system employing gold electrodes at 0% strain ( Supplementary Fig. S15 ). We also show that the conductive path can be maintained on non-planar substrates ( Fig. 4e,f ), where conformal wrapping can occur easily owing to the low-bending modulus, thin form, and highly elastic properties. LED arrays with various colours (red, green, orange) can be realized on hemispherical substrates using this approach ( Fig. 4g ). The methods and the collective set of results reported here represent concepts for realizing materials and structures with much higher levels of stretchability and conductivity compared with conventional methods. A critical component to this work is the identification of the mechanism responsible for the enhanced stretchability beyond intrinsic limits in 3D nanostructured materials. The strategy is agnostic to the particular elastomer formulation. The most important outcome, then, is the improvement in stretchability for the elastomer studies, rather than an absolute comparison against other materials. A remaining technical barrier in application of the technology is the fabrication of thicker 3D structures. Exploring other materials, such as metal or ceramic, represents another promising direction for future work. Preparation of silicon masters A bottom antireflective coating (K-131, Dongin Semichem) with a thickness of ~58 nm was formed on an 8-inch silicon wafer using a track system (K Spin8, SEMES). Then, a thin photoresist (LX-429, Dongjin Semichem) film with a thickness of ~400 nm was spincoated and exposed at 22 mJ cm −2 through a pre-patterned ultraviolet reticle using a KrF (248 nm) scanner (NSR-S203B, Nikon). After developing the exposed film with developer (DPD 200, Dongjin Semichem) for 60 s, bottom antireflective coating etching was performed with a deep silicon etcher (TCP-9400, Lam Research) using CF 4 gas and a flow rate of 100 s.c.c.m., at a main power of 250 W with a bottom power of −250 W, at 7 mTorr. Subsequently, silicon etching formed relief structures with depths of ~400 nm, using Cl 2 gas with a flow rate of 72 s.c.c.m., HBr gas with a flow rate of 180 s.c.c.m., O 2 gas with a flow rate of 7 s.c.c.m., at a main power of 300 W with a bottom power of −225 W. Finally, the residual photoresist on the top of silicon masters was removed using a photoresist stripper (DAS2000, PSK). Preparation of conformal phase masks The silicon master was pre-treated by perfluorinated trichlorosilane (T2492, United Chemical Technologies) vapour in a dessicator to prevent strong adhesion between the master and the silicone elastomer. A bilayer structure of two different types of PDMS was used to replicate nanostructures against the master. A hard modulus PDMS (~10 MPa) (h-PDMS) (VDT-731, HMS-301, Gelest) was directly spin-coated onto the master at 1,000 r.p.m. for 30 s. Next, continuous spinning at 500 r.p.m. for 30 min yielded partially crosslinked h-PDMS with a flat surface. Subsequently, a relatively soft PDMS (~2 MPa) (s-PDMS) (Sylgard 184, Dow Corning) was poured on top of the first layer to facilitate manipulation of the resulting soft, conformable phase mask. Fully curing the bilayer PDMS for 1 day at room temperature and then peeling it away from the master completed the process. Preparation of photoresists on substrates A glass substrate (G480-15, ProSciTech) was oxygen-plasma treated with a flow rate of 45 s.c.c.m., a pressure of 40 mTorr, and a power of 60 W for 2 min using a plasma treatment system (CUTE-MP, Femtoscience). Thin AZ 9260 (~5 μm) was pre-coated on the cleaned substrate as a releasing layer to enable delamination of free-standing thin films of PDMS from the substrate during the template removal step. The releasing layer was hard-baked on at 110 °C for 5 min. Subsequently, relatively thick photoresist (~12 μm) was spin-coated on the releasing layer at a spin-speed of 2,000 r.p.m. for 30 s. The resist-coated substrate was then soft-baked at 100°C for 5 min. Fabrication of 3D templates by Proximity-field nanoPatterning (PnP) The optical set-up for PnP includes a pulsed, passively Q-switched Nd:YAG microchip laser (355 nm, 14 mW, Teem Photonics) with a beam expander and a collimator as a coherent ultraviolet light source. Placing the PDMS phase mask on the surface of the AZ 9260 film leads to intimate atomic scale, conformal contact driven by Van der Waals forces without any pressure. Passing collimated light through the mask generates a complex 3D intensity distribution in the AZ 9260 film. The exposure doses ranged from 50 to 450 mJ cm −2 . The exposed regions were then dissolved away using a water-based developer (AZ 400 K, 1:3 dilution of buffered KOH, Clariant) and rinsed by de-ionized water. Fabrication of 3D PDMS by templating processes A s-PDMS prepolymer was prepared by mixing the base component and the curing agent in 10:1 ratio. The mixture was degassed in a small dessicator for 1 h to completely remove air bubbles, and it was poured onto the oxygen-plasma treated 3D template. Infiltrated sample was degassed again in a dark dessicator for 1 h to ensure that prepolymer successfully filled into the porous nanonetwork of the 3D template. Spin-casting with various spin-speeds ranging from 1,000 to 7,000 r.p.m. enabled a controlled process for levelling an upper residual layer consisting of solid PDMS. After curing the s-PDMS at 60 °C for 2 h in a clean oven, a second flood exposure allowed the original template and the releasing layer to be removed with organic solvents. A free-standing PDMS film, which was inversely replicated from the 3D polymer template, floated onto a developer bath (AZ 400 K, 1:4 dilution of buffered KOH, Clariant) as a result of dissolving the releasing layer. Scooping up this film using a thick, conformal PDMS slab successfully yielded a back-supported thin, 3D porous sheet of PDMS. Fabrication of stretchable conductors The stretchable conductor was prepared by infiltrating eutectic gallium–indium alloy (EGaIn, Sigma-Aldrich) into 3D PDMS. Two samples of 3D PDMS with narrow strips of solid PDMS at the edges, supported by thick PDMS slabs with releasing layers (AZ 5214-E, Clariant), were oxygen-plasma treated at a flow rate of 45 s.c.c.m., pressure of 40 mTorr, and power of 60 W for 120 s. EGaIn was dropped and spread on the top of the plasma-treated 3D PDMS. The sample was degassed in a dessicator overnight to squeeze EGaIn into the porous channel of 3D PDMS. After pressing on the top of EGaIn-filled 3D PDMS with a PDMS block and the sample was spun-cast at 8,000 r.p.m. to reduce residual EGaIn remaining outside the pores. To ensure successful filling, the above infiltration steps were repeated several times. Finally, two samples prepared with this method were sealed together. Weakly pressing the marginally solid PDMS for few seconds enables perfect sealing of EGaIn. Removal of releasing layers by developer yielded enclosed stretchable conductors. Optical modelling The 2D calculation of the intensity distribution of the ultraviolet light in the photoresist film, through the PDMS phase mask, was conducted using a finite elements modelling software (COMSOL Multiphysic 3.5, COMSOL). The 3D reconstructed images of the structures formed by PnP were simulated using rigorous coupled wave analysis software (GSOLVER V4.20, Grating Solver Development). Characterization The structural details of positive-tone templates and 3D PDMS were investigated by field-emission scanning electron microscopy (S-4800, Hitachi) operated at an accelerating voltage of 5–10 kV. Absorption measurements of AZ 9260 films were performed using a UV-VIS spectrometer (UV-310PC, Shimadzu). The mechanical tensile tests were conducted using a customized flexible tester and a commercial microload test system (UNITECH). The electrical conductivity of stretchable conductors was measured by a four-point probe system. All results appearing in the text about mechanical properties and conductivity were based on average values of many (>10) samples tested. How to cite this article: Park, J. et al . Three-dimensional nanonetworks for giant stretchability in dielectrics and conductors. Nat. Commun. 3:916 doi: 10.1038/ncomms1929 (2012).